Chemical synthesis of lactic acid from cellulose catalysed by lead(II) ions in water The direct transformation of cellulose, which is the main component of lignocellulosic biomass, into building-block chemicals is the key to establishing biomass-based sustainable chemical processes. Only limited successes have been achieved for such transformations under mild conditions. Here we report the simple and efficient chemocatalytic conversion of cellulose in water in the presence of dilute lead(II) ions, into lactic acid, which is a high-value chemical used for the production of fine chemicals and biodegradable plastics. The lactic acid yield from microcrystalline cellulose and several lignocellulose-based raw biomasses is >60% at 463 K. Both theoretical and experimental studies suggest that lead(II) in combination with water catalyses a series of cascading steps for lactic acid formation, including the isomerization of glucose formed via the hydrolysis of cellulose into fructose, the selective cleavage of the C3–C4 bond of fructose to trioses and the selective conversion of trioses into lactic acid. There is a strong incentive to produce chemicals and fuels from renewable biomass resources to reduce the reliance on diminishing fossil resources [1] , [2] . Although the conventional biological process, typically the fermentation of biomass-based carbohydrates, possesses some advantages, a chemocatalytic process provides opportunities to increase the process efficiency because the catalysts and the operation conditions can be readily engineered and optimized. Furthermore, chemocatalysis may allow the direct transformation of biomass feedstocks other than monosaccharides or oligosaccharides into chemicals in a one-pot process by designing multifunctional catalytic systems. Many studies have been devoted to establishing the basis for the conversion of biomass-based carbohydrates into liquid fuels and chemicals via platform molecules, such as 5-hydroxymethylfurfural (HMF) [3] , [4] , [5] , [6] . However, less attention has been paid to developing chemocatalytic routes for the production of building-block chemicals directly from biomass [7] , [8] , [9] , [10] . Lignocellulosic biomass is expected to be the most promising renewable biomass feedstock owing to its wide abundance [1] . The efficient transformation of cellulose, the main component of lignocellulosic biomass, into chemicals is essential for the utilization of lignocellulosic biomass as a chemical feedstock. The high-temperature gasification of cellulose to synthesis gas, which can be used for the synthesis of methanol or hydrocarbons, is limited by a high-energy requirement and low selectivity [11] . The hydrolysis of cellulose by cellulase occurs at ambient temperatures [12] , but this high-cost process is currently impractical for large-scale production of glucose. The transformation of cellulose in ionic liquids, which can dissolve cellulose, has received much attention [13] , but ionic liquids are expensive. The chemocatalytic conversion of cellulose into chemicals in water under mild conditions is an ideal but highly challenging route [14] , [15] . Moderate success has been achieved for the hydrogenolysis of cellulose into polyols (for example, ethylene and propylene glycols of commercial interest) [16] , [18] . However, the consumption of hydrogen is required in these reactions. There are few systems capable of catalysing the transformation of cellulose directly into high-value chemicals in water without the consumption of hydrogen. Lactic acid is an important building-block chemical widely used in the food, pharmaceutical, cosmetic and chemical industries. In particular, lactic acid has received much attention as a monomer for the production of biodegradable plastics [8] , [9] , [10] , [19] , [20] . Currently, lactic acid is primarily produced by the fermentation of glucose. However, this biological process is not applicable directly to cellulose, and the pre-hydrolysis of cellulose to glucose is required. Due to the growing demand for lactic acid, this biocatalytic route may have important roles in industry. At the same time, the development of novel chemocatalytic processes for the production of lactic acid from biomass has also attracted much attention in recent years [21] . The chemical conversion of carbohydrates to lactate salts with low yields (<30%) does proceed in alkaline medium (for example, NaOH) at temperatures of ~573 K [22] . The harsh reaction conditions, limited yields and consumption of a stoichiometric amount of base hinder the commercialization of this process. Recent reports disclosed that Sn(IV)-beta and Sn(IV) grafted on a mesoporous carbon–silica composite could catalyse the conversion of carbohydrates, such as glucose, fructose and sucrose, in an alcohol medium into alkyl lactate [8] , [9] . Although promising, these Sn(IV)-based catalysts are limited to the transformation of mono or disaccharides. Herein, we report for the first time that lactic acid can be directly produced from cellulose with high efficiency by a simple chemocatalytic system. The system is composed of a diluted metal ion (i.e., Pb(II)) in water. The chemistry of this system has been clarified through comprehensive theoretical studies as well as experimental validation. We have demonstrated that simple Pb(II) in combination with water can accomplish complicated cascade reactions for the transformation of cellulose to lactic acid. Catalytic performance of Pb(II) for cellulose conversion We discovered that cellulose could be converted directly into lactic acid in hot water by simply adding a metal cation. 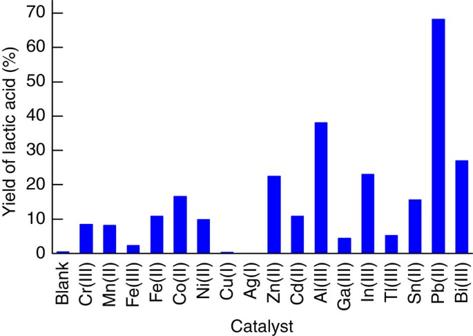Figure 1: Catalytic performance of metal cations for the conversion of cellulose to lactic acid. Reaction conditions: metal cation, 0.14 mmol; ball-milled cellulose, 0.10 g (glucose unit: 0.62 mmol); N2, 3 MPa; H2O, 20 ml; temperature, 463 K; reaction time, 4 h. Figure 1 shows that an outstanding yield of lactic acid (68%) has been attained in the presence of diluted Pb(II) with a concentration of 7 mmol dm −3 (mM) for the conversion of ball-milled cellulose (crystallinity=33%, Supplementary Fig. S1 ) after 4 h at 463 K. In addition, glucose, fructose and organic acids, such as glycolic acid and levulinic acid, were also formed but with lower yields ( Supplementary Note S1 ). Other cations, including Al(III), Bi(III), In(III) and Zn(II), with d 10 or d 10 s 2 electronic configuration also catalysed the conversion of the ball-milled cellulose into lactic acid with yields of >20%. In most cases, metal nitrates were employed in our experiments, and we confirmed that the counter anions did not exert significant influences on the catalytic performance ( Supplementary Table S1 ). Figure 1: Catalytic performance of metal cations for the conversion of cellulose to lactic acid. Reaction conditions: metal cation, 0.14 mmol; ball-milled cellulose, 0.10 g (glucose unit: 0.62 mmol); N 2 , 3 MPa; H 2 O, 20 ml; temperature, 463 K; reaction time, 4 h. Full size image We investigated the effect of the concentration of Pb(II) on the transformation of the ball-milled cellulose. In the absence of Pb(II), the ball-milled cellulose could also be converted in water at 463 K to yield glucose and HMF as the main products. No lactic acid was formed. We speculate that the H 3 O + ions, which are reversibly generated in hot water owing to the increased ionization constant of water at higher temperatures [23] , [24] , can catalyse the hydrolysis of the ball-milled cellulose to glucose. HMF can be formed by the dehydration of fructose [3] , [4] , [25] , which is an isomer of glucose. The presence of Pb(II) decreased the yields of glucose and HMF, and resulted in the formation of lactic acid ( Supplementary Fig. S2 ). The yield of lactic acid increased steeply with the concentration of Pb(II) and reached ~50% at a Pb(II) concentration of 0.7 mM. The turnover number (TON) for the lactic acid formation evaluated at this concentration of Pb(II) was 22. Further increases in the concentration of Pb(II) slightly increased the yield of lactic acid, and a plateau of ~70% was attained. We performed the conversion of cellulose with different quantities in 100 ml water. A lactic acid yield of 55% could be obtained for a cellulose quantity of 2.5 g ( Supplementary Table S2 ). The molar ratio of the glucose unit in cellulose to Pb(II) was 25 at this point providing a TON of 14. An increase in the molar ratio of the glucose unit in cellulose to Pb(II) to 300 by decreasing the amount of Pb(II) provided a lactic acid yield of 34% and a TON of 102. However, a further increase in the quantity of cellulose to 5.0 g significantly decreased the yield of lactic acid owing to poor mechanical agitation and the formation of humin possibly via the dehydration of carbohydrate intermediates resulting from the increased Brønsted acidity of the solution. As expected, the conversion of microcrystalline cellulose (crystallinity=85%) became more difficult. In the absence of Pb(II), HMF and glucose were also obtained as the main products, but their yields were only ~9 and 4% even after 15 h of reaction at 463 K ( Supplementary Fig. S3 ). The presence of Pb(II) accelerated the conversion of microcrystalline cellulose, and a lactic acid yield of 62% was attained after 15 h of reaction at 463 K. Therefore, Pb(II) ions had significant roles both in directing the reaction towards the formation of lactic acid and in enhancing the conversion of microcrystalline cellulose. We further clarified that the lactic acid product enhanced the conversion of cellulose. The intentional addition of lactic acid into the reaction system significantly shortened the time required to achieve a lactic acid yield of ~60% ( Supplementary Fig. S4 ), which clearly indicated the autocatalytic function of lactic acid (p K a of 3.66 at 298 K) in the hydrolysis of cellulose. Conversions of other biomasses and raw biomasses The present catalytic system is applicable to the transformation of other biomasses, such as starch and inulin, which are polymers of glucose and (fructose+glucose) ( Supplementary Table S3 ). The yields of lactic acid from starch and inulin reached 68% and 73%, respectively, after 2 h of reaction at 463 K ( Supplementary Table S4 ). We also examined the direct transformations of several lignocellulose-based non-purified raw biomasses including sugar bagasse, couch grass and bran (see Supplementary Table S3 for compositions) in the presence of Pb(II) and obtained lactic acid yields of ≥66% based on the amount of C 6 and C 5 monosaccharide units contained in these biomasses ( Supplementary Table S4 and Supplementary Note S2 ). For the conversions of inulin, starch and the raw biomasses (sugar bagasse, couch grass and bran), the use of a larger quantity (2.5 g in 100 ml water) resulted in lactic acid yields of ≥41% based on the amount of C 6 and C 5 monosaccharide units contained in these biomasses ( Supplementary Table S5 ). In addition, we performed the separation and recovery of Pb(II) from the reaction system and found that all of the Pb(II) ions in the reaction solution could be recovered simply by using a cationic exchanging resin (Amberlite IR-120 resin) ( Supplementary Note S3 ). Reaction mechanism and catalytic function of Pb(II) To gain insights into the reaction pathways, we performed the conversion of glucose and fructose, which are two possible monosaccharide intermediates. In the absence of Pb(II), HMF was the main product in both cases ( Fig. 2a ). The presence of Pb(II) increased the conversion of either glucose or fructose, especially at lower temperatures (≤433 K), and switched the main product from HMF to lactic acid ( Fig. 2b and d ). The lactic acid yields reached 71% and 74% for the conversions of glucose and fructose at 443 and 463 K, respectively. Pb(II) also enhanced the conversion of glucose to fructose at ≤433 K ( Fig. 2b ). A detailed time-course analysis for the conversion of glucose at 423 K in the presence of Pb(II) indicated that fructose was the intermediate for the conversion of glucose to lactic acid ( Supplementary Fig. S5 ). These results suggest that the reaction proceeds via the reaction pathways shown in Fig. 3 . Pb(II) catalyses both the isomerization of glucose to fructose and the conversion of fructose to lactic acid. 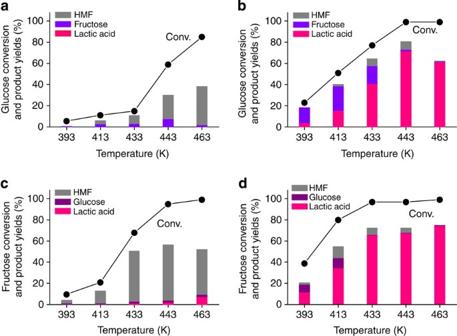Figure 2: Conversion of glucose and fructose in the absence and presence of Pb(II). (a) Glucose conversion in the absence of Pb(II). (b) Glucose conversion in the presence of Pb(II). (c) Fructose conversion in the absence of Pb(II). (d) Fructose conversion in the presence of Pb(II). Conv., conversion. Reaction conditions: Pb(II), 0.14 mmol; glucose, 0.51 mmol; fructose, 0.56 mmol; H2O, 20 ml; N2, 3 MPa; reaction time, 2 h. Figure 2: Conversion of glucose and fructose in the absence and presence of Pb(II). ( a ) Glucose conversion in the absence of Pb(II). ( b ) Glucose conversion in the presence of Pb(II). ( c ) Fructose conversion in the absence of Pb(II). ( d ) Fructose conversion in the presence of Pb(II). Conv., conversion. 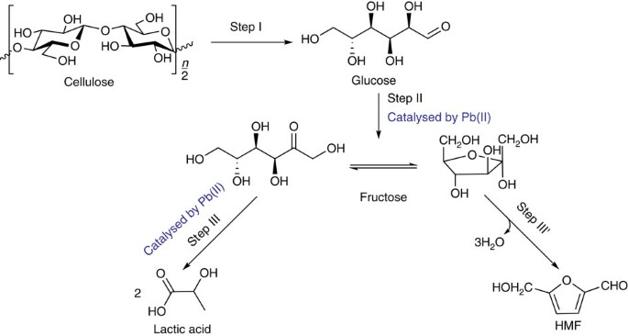Figure 3: Reaction pathways. Reaction pathways for the conversion of cellulose into lactic acid and HMF in the presence and absence of Pb(II) in water. Reaction conditions: Pb(II), 0.14 mmol; glucose, 0.51 mmol; fructose, 0.56 mmol; H 2 O, 20 ml; N 2 , 3 MPa; reaction time, 2 h. Full size image Figure 3: Reaction pathways. Reaction pathways for the conversion of cellulose into lactic acid and HMF in the presence and absence of Pb(II) in water. Full size image We conducted theoretical computations for the conversion of glucose to lactic acid using a cluster-continuum model to elucidate the reaction mechanism and the catalytic function of Pb(II). The computational approach adopted in the current study has been verified to be practicable for chemical reactions in aqueous solutions [26] , [27] . Our computational results are displayed in Fig. 4 and Table 1 , and the details are summarized in the Supplementary Information ( Supplementary Figs S6–S33 and Supplementary Tables S6–S9 ). In brief, the conversion of glucose to lactic acid can be roughly divided into the following three stages: (i) the isomerization of glucose to fructose ( 1 → 3 ), (ii) the retro-aldol fragmentation of fructose producing two C 3 intermediates or trioses ( 3 → 4 + 5 ) and (iii) the isomerization of these trioses ( 4 ↔ 5 → 11 ) into lactic acid ( Fig. 4 ). 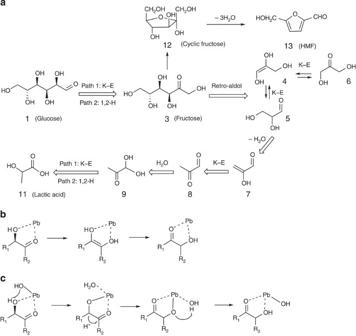Figure 4: Reaction mechanism. (a) Proposed reaction mechanism based on theoretical computations for the conversion of glucose to lactic acid in water. (b) Path 1 for the isomerization of glucose or trioses: K–E (i.e., consecutive keto–enol tautomerization) via the Pb(II) model. (c) Path 2 for the isomerization of glucose or trioses: 1,2-H (i.e., 1,2-hydride shift) via the Pb(II)–OH model. The calculated activation Gibbs energies and Gibbs free energies for the key steps are displayed inTable 1. Figure 4: Reaction mechanism. ( a ) Proposed reaction mechanism based on theoretical computations for the conversion of glucose to lactic acid in water. ( b ) Path 1 for the isomerization of glucose or trioses: K–E (i.e., consecutive keto–enol tautomerization) via the Pb(II) model. ( c ) Path 2 for the isomerization of glucose or trioses: 1,2-H (i.e., 1,2-hydride shift) via the Pb(II)–OH model. The calculated activation Gibbs energies and Gibbs free energies for the key steps are displayed in Table 1 . Full size image Table 1 Activation Gibbs energy and Gibbs free energy values. Full size table For the isomerization of glucose to fructose, we performed computations for two possible paths (that is, the consecutive keto–enol tautomerization (denoted as K–E) and the 1,2-hydride shift (denoted as 1,2-H) paths) [28] , [29] , [30] . The activation Gibbs energies (Δ G ≠ ) obtained for these two paths were 24.1 and 32.8 kcal mol −1 in aqueous solution without the Pb(II) catalyst ( Supplementary Table S6 and Supplementary Fig. S10 ). This result suggests that the consecutive keto–enol tautomerization path is more favourable in the non-catalytic reaction. The presence of Pb(II) decreased the activation Gibbs energy for this path to 22.0 kcal mol −1 ( Supplementary Table S8 ). A Sn(IV)–OH species had been proposed to be responsible for the Sn-beta-catalysed isomerization of glucose to fructose [29] , [30] . Our computation provided a low energy barrier (Δ G ≠ =3.6 kcal mol −1 ) for the transformation of Pb(II) to Pb(II)–OH in water ( Supplementary Fig. S19 ). Many studies have demonstrated the formation of Pb(II)–OH in an aqueous solution of Pb(II) ( Supplementary Note S4 ) [31] , [32] , [33] , [34] . Our experimental studies using Fourier-transform ion cyclotron resonance mass spectrometry, which is a very powerful technique for the structural determination of new compounds with ultra-high mass resolution and accuracy [35] , [36] , provided further evidence for the existence of the Pb(II)–OH species in the Pb(II) aqueous solution ( Supplementary Fig. S34 ). When Pb(II)–OH is assumed to be the active species instead of Pb(II), the calculation indicates that the activation Gibbs energy for the 1,2-hydride shift path (Δ G ≠ =19.5 kcal mol −1 ) is lower than that for the keto–enol tautomerization path (Δ G ≠ =22.0 kcal mol −1 ) ( Supplementary Fig. S24 and Supplementary Table S8 ). Using deuterium-labelled glucose (glucose-D2) as the substrate, we experimentally confirmed that the isomerization of glucose into fructose primarily proceeded via the 1,2-hydride shift mechanism in the presence of the lead catalyst ( Supplementary Fig. S35 ). These results suggest the role of the Pb(II)–OH species in the isomerization of glucose to fructose. The conversion of the trioses formed from the cleavage of the C–C bond of fructose undergoes several isomerization steps as well as dehydration and hydration to form lactic acid ( 5 → 11 ). Our calculations suggest that the 1,2-hydride shift is also a preferential path for the isomerization of 1,1-dihydroxy-acetone to lactic acid ( 9 → 11 ) ( Supplementary Fig. S33 ), which is the most difficult step in the conversion of trioses to lactic acid. In addition to the isomerization reactions, the retro-aldol fragmentation of fructose into trioses (that is, glyceraldehyde ( 5 ) and enediol intermediate ( 4 )) is a crucial step. In the absence of Pb(II), our calculations indicate that the activation Gibbs energy for this step is 32.8 kcal mol −1 ( Supplementary Fig. S11 ), which is a highly energy demanding step in the non-catalytic transformation of glucose to lactic acid ( Table 1 ). In comparison with the retro-aldol fragmentation, the dehydration of fructose into HMF ( 3 → 13 ) proceeds with a lower energy barrier in the absence of Pb(II) ( 3 → 12 : Δ G ≠ =22.0 kcal mol −1 , 12 → 13 : Δ G ≠ =29.1 kcal mol −1 ; Supplementary Fig S17 and Supplementary Table S7 ). The presence of Pb(II) significantly reduces the activation Gibbs energy for the retro-aldol fragmentation from 32.8 to 22.4 kcal mol −1 ( Supplementary Table S9 ). The activation Gibbs energy for this step increases slightly (Δ G ≠ =24.4 kcal mol −1 ) when Pb(II)–OH is assumed to be the active species ( Supplementary Fig. S29 ). Therefore, it becomes quite clear that Pb(II) has a crucial role in the cleavage of the C–C bond of fructose. Without Pb(II), the dehydration of fructose to HMF would preferentially proceed owing to the relatively lower energy barrier for the dehydration compared with that for the retro-aldol fragmentation. Our tandem mass spectrometry studies provided experimental evidence for the catalytic function of Pb(II) in the retro-aldol reaction. In the mass (MS) and the tandem mass (MS/MS) spectra, we observed the species of the Pb–fructose complex and the fragment formed via the cleavage of the C3–C4 bond in fructose coordinated to Pb(II) ( Supplementary Fig. S36 ). Only the fragments from the dehydration of fructose were detected in the MS and the MS/MS spectra in the absence of Pb(II) ( Supplementary Fig. S37 ). Our computational results displayed in Table 1 reveal that the presence of Pb(II) also significantly decreases the activation barrier for reaction step 9 → 11 , which is the most difficult step in the conversion of trioses to lactic acid. In addition, we performed experimental studies on the conversion of trioses (that is, glyceraldehyde ( 5 ), dihydroxyacetone ( 6 ) and pyruvaldehyde ( 8 )) at 463 K in aqueous solutions. For the conversion of all of these trioses in the presence of Pb(II), lactic acid was produced with high yields (≥91%), while the absence of Pb(II) led to significantly lower lactic acid yields (≤18%) ( Supplementary Table S10 ). This suggests that our Pb(II) catalyst also has a role in the conversion of trioses to lactic acid. We discovered a simple and highly efficient homogeneous catalyst for the direct transformation of cellulose into lactic acid in an aqueous solution. The system containing diluted Pb(II) in water not only catalyses the conversion of ball-milled cellulose, as well as glucose and fructose, to lactic acid with high yields (~70%) but also is efficient for the conversion of microcrystalline cellulose (lactic acid yield, ~60%). The system is also applicable to the transformation of lignocellulose-based raw biomasses without pretreatment. To the best of our knowledge, this is the first report to demonstrate the production of lactic acid with considerable yields (>50%) from cellulose. We have clarified that the chemistry of the present system involves multistep cascade reactions including the hydrolysis of cellulose to glucose, the isomerization of glucose to fructose, the retro-aldol fragmentation of fructose to trioses and the conversion of trioses to lactic acid. While the dehydration of fructose to HMF primarily occurs in the absence of Pb(II), the presence of Pb(II) shifts the main reaction route to the formation of lactic acid. Our computational results agree well with the experimental findings and provide a basis for understanding the remarkable catalytic role of Pb(II). In particular, the presence of Pb(II) significantly decreases the activation barrier for the retro-aldol fragmentation of fructose changing the main reaction route from the formation of HMF to the formation of lactic acid. A detailed reaction path analysis reveals that the C–C bond cleavage of fructose is triggered by the proton transfer from the C4–OH to C2=O ( Supplementary Fig. S27 ). Our calculation suggests that the coordination of Pb(II) to the oxygen atoms of fructose increases the positive charges on the H atom of the C4–OH ( Supplementary Figs S11, S27 and S28 ). This indicates that Pb(II) enhances the acidity of the C4–OH, thereby facilitating the proton transfer and the C–C bond cleavage in the retro-aldol reaction. In comparison with other metal ions, the larger size (radius of Pb(II)=119 pm) and closed shell of Pb(II) may lead to it being better coordinated by the oxygen atoms of fructose. This may allow Pb(II) to mediate the initial proton transfer more effectively in the above step. In addition, the lone electron pair (6s 2 ) of Pb (II) may promote the proton transfer [31] , [32] contributing to its outstanding catalytic performances. These features may explain why Pb(II) demonstrates better catalytic performances for the formation of lactic acid than many other metal ions ( Fig. 1 ). Our computational studies further suggest that the Pb(II)–OH species in the aqueous solution may primarily contribute to catalysing the isomerization of glucose to fructose and that of the trioses to lactic acid via the 1,2-hydride shift mechanism. We have experimentally demonstrated the generation of Pb(II)–OH in the Pb(II) aqueous solution. Future experimental studies are needed to clarify the interaction of the Pb(II)–OH species with the substrate under reaction conditions. In addition to Pb(II) and Pb(II)–OH species, water molecules and the reversibly generated protons in hot water also have roles in some of the steps. Furthermore, lactic acid autocatalyzes the hydrolysis of microcrystalline cellulose. It is encouraging that simple Pb(II) in combination with water can accomplish such complicated cascade reactions. It is important to note that the toxicity of Pb(II) should be considered before the practical application of the present catalytic system for the production of lactic acid from cellulose. We have demonstrated that Pb(II) can be separated and recovered by using a cationic exchanging resin, but the separation and recovery of Pb(II) would increase the process cost. In addition, because of the difficulties in separating lactic acid from the aqueous solution containing the byproducts, including glucose, fructose and other organic acids, and its subsequent purification, the product selectivity should be further improved. Nevertheless, the results and insights obtained in the current work are quite encouraging and can inspire further design of more environmental friendly and more efficient catalytic systems for the transformation of cellulose to lactic acid in water. As a first step, we have attempted to use the combination of dual or multiple cations for the conversion of glucose, because the most suitable catalysts for different steps in the cascade reactions for converting glucose to lactic acid may be different. Very recently, we found that a dual-cation system, which was composed of Al(III) and Sn(II) with a molar ratio of 1/1, provided a lactic acid yield of 81% from glucose after 2 h at 463 K, which is a higher yield than that obtained with Pb(II) (71%). The conversion of ball-milled cellulose with the Al(III)–Sn(II) combination afforded a lactic acid yield of 66% after a reaction at 463 K for 4 h, which is comparable to that obtained with Pb(II). Further improvements can be expected through clarification of the roles of the different catalytic components in each step of the cascade reactions from cellulose to lactic acid and further optimization of the dual- or multicomponent catalytic systems. Materials and general methods The microcrystalline cellulose was purchased from Alfa-Aesar. The chemicals primarily used in this work were as follows: D -(+)-glucose (99.5%, Alfa-Aesar), D -fructose (99%, Alfa-Aesar) and Pb(NO 3 ) 2 (99%, Alfa-Aesar). The ball-milled cellulose was obtained by ball-milling the purchased microcrystalline cellulose at 60 r.p.m. on a SFM-1 Desk-top planetary ball miller (MTI Corporation) for 48 h. The crystallinity was estimated from the X-ray diffraction patterns of the cellulose samples [37] . X-ray diffraction patterns were collected on a Panalytical X’pert Pro diffractometer using Cu K α radiation (40 kV, 30 mA). Fourier-transform ion cyclotron resonance mass spectrometry measurements were performed on a Bruker APEX IV 7.0T Fourier-transform ion cyclotron resonance mass spectrometer in positive ion mode equipped with an external electrospray ionization source. Pb(NO 3 ) 2 was dissolved in water to obtain a concentration of ~0.15 mmol l −1 . This solution was electrosprayed from a capillary biased at 4,400 V. The scan range of m/z was from 100 to 600. An accuracy of m/z of 1 × 10 −5 was achieved. 1 H NMR spectra were recorded on a Bruker Avance II 400 MHz instrument operating at 400 MHz. All of the experiments were conducted in D 2 O with chemical shifts reported in parts per million downfield from sodium 3-(trimethylsilyl)-1-propanesulphonate (DSS). The tandem mass spectrometry measurements were performed on an Esquire 3000 Plus mass spectrometer equipped with an electrospray ionization source. The ionization was performed under normal electrospray conditions (flow rate: 4 μl min −1 , 4.5 kV, dry temperature: 493 K). A collision energy between 0.2 and 0.8 V p–p was employed for each collision-induced dissociation stage (in each case, the precursor beam attenuation was set between 0 and 10%), and a mass range between 2 and 4 Da was isolated before the collision-induced dissociation experiment (the isolation width was increased with the number of multiple stage experiments to maintain as many ions as possible in the trap). Catalytic reaction The conversions of cellulose, hexose and triose intermediates, and other biomasses were performed in a batch-type Teflon-lined stainless-steel autoclave. For example, for the conversion of cellulose, the catalyst and the powdery cellulose sample were added to the reactor that had been pre-charged with H 2 O. After the introduction of N 2 at a pressure of 3 MPa, the reactor was placed in an oil bath. After the system reached the reaction temperature (typically 463 K), the reaction was initiated by vigorous stirring. After a fixed time, the reaction was quickly terminated by cooling the reactor to room temperature in cold water. The liquid products were analysed by high-performance liquid chromatography (HPLC, Shimazu LC-20A) equipped with an RI detector and a Shodex SUGARSH-1011 column (8 × 300 mm 2 ) using a dilute H 2 SO 4 aqueous solution as the mobile phase. The yields of the main products, such as lactic acid, glucose, fructose and HMF, are primarily displayed herein, and the details of the other byproducts are described in Supplementary Note S2 . We performed the same experiment at least in triplicate for each run, and the relative error was <3%. The high-performance liquid chromatography quantification was further validated via a titration method [38] . Theoretical computation All of the calculations were performed with the Gaussian 09 software package. The geometries of all of the transition states, reactants and intermediates involved in the reaction were fully optimized using a hydrated cluster in conjunction with the continuum solvation model of SMD at the B3LYP/6-31G(d) level of theory (the LanL2DZ-ECP basis set was employed for Pb). Harmonic frequency calculations were performed at the equilibrium geometries to confirm first-order saddle points and local minima on the potential energy surfaces, and to estimate the zero-point energy, as well as the thermal and entropic corrections, at 298.15 K and 1 atm. The correlation between the stable structures and the transition states was verified by analysing the corresponding imaginary frequency mode, as well as by limited intrinsic reaction coordinate calculations. The relative energies of the B3LYP/6-31G(d)-optimized structures were further refined by single-point calculations at the B3LYP/6-311++G(d,p) level (the polarized LANL2DZdp ECP basis set was employed for Pb) with inclusion of solvent effects. Natural bond orbital analyses at the B3LYP/6-311++G(d,p) level were performed to determine the atomic charge populations. For estimation of the Gibbs free energy, direct calculations in combination with frequency analysis in solution were performed, which has been verified to be a correct and practical approach [39] especially when liquid-phase and gas-phase structures differed significantly or when the stationary points present in the liquid solution could not survive in the gas phase. The B3LYP method was compared with several other popular density functional theoretical methods, including B3PW91, B97-D, M06, X3LYP and M06-2X, for the isomerization of glucose to its enol form, and B3LYP was found to be adequate for the present mechanistic study. In addition to 298.0 K, thermal corrections were also assessed at 463.0 K to explore the temperature effect on the Gibbs free energy, and the temperature effect was not remarkable here. How to cite this article: Wang, Y. et al. Chemical synthesis of lactic acid from cellulose catalysed by lead(II) ions in water. Nat. Commun. 4:2141 doi: 10.1038/ncomms3141 (2013).